Development of a novel selective inhibitor of the Down syndrome-related kinase Dyrk1A Dyrk1A (dual-specificity tyrosine-(Y)-phosphorylation-regulated kinase 1A) is a serine/threonine kinase essential for brain development and function, and its excessive activity is considered a pathogenic factor in Down syndrome. The development of potent, selective inhibitors of Dyrk1A would help to elucidate the molecular mechanisms of normal and diseased brains, and may provide a new lead compound for molecular-targeted drug discovery. Here, we report a novel Dyrk1A inhibitor, INDY, a benzothiazole derivative showing a potent ATP-competitive inhibitory effect with IC 50 and K i values of 0.24 and 0.18 μM, respectively. X-ray crystallography of the Dyrk1A/INDY complex revealed the binding of INDY in the ATP pocket of the enzyme. INDY effectively reversed the aberrant tau-phosphorylation and rescued the repressed NFAT (nuclear factor of activated T cell) signalling induced by Dyrk1A overexpression. Importantly, proINDY, a prodrug of INDY, effectively recovered Xenopus embryos from head malformation induced by Dyrk1A overexpression, resulting in normally developed embryos and demonstrating the utility of proINDY in vivo . Dyrk1A (dual-specificity tyrosine-(Y)-phosphorylation-regulated kinase 1A) is a serine/threonine kinase that is essential for maintaining the normal development and function of the brain; it is expressed in fetal as well as adult brains, where it phosphorylates myriad proteins and thereby regulates their functions [1] , [2] . The physiological importance of Dyrk1A has recently been highlighted by its proposed relation with the pathogenesis of Down Syndrome (DS) [2] . DS is a congenital genetic disorder that appears in 1 in every 733 births in the United States [3] . DS is caused by a complete or partial trisomy of chromosome 21, and is characterized by systemic manifestations including mental retardation, cardiovascular anomalies, craniofacial dysmorphology, malignant neoplasms such as acute myoblastic leukaemia and recurrent infections [2] , [4] . The genetically complex nature of the disease has hindered development of effective drugs [4] . xDyrk1A resides within the so-called Down Syndrome Critical Region (DSCR) of human chromosome 21 (refs 5 , 6 , 7 ), a genomic region that has an important role in DS manifestations, if indeed it is not solely responsible for the pathogenesis of DS [8] , [9] . The extra copy of the Dyrk1A gene in DS indeed results in a 1.5-fold increase in the Dyrk1A product at both the protein and activity levels in the brain [10] , [11] , [12] , [13] . Importantly, several studies using different lines of transgenic mice have revealed that overexpression of Dyrk1A alone is sufficient to induce brain morphology alterations, as well as neurological and motor disorders that may be reminiscent of the learning deficits and altered motor skill acquisition seen in patients with DS [14] , [15] , [16] , [17] , [18] , [19] , [20] , [21] . The events downstream of Dyrk1A in these disease models are not yet completely understood; however, aberrant phosphorylation of NFATc transcription factors, components of the calcineurin/NFAT (nuclear factor of activated T cell) signalling pathway, is proposed to have a role in the pathogenesis of DS. Arron et al . [22] reported that Nfatc1 −/− -knockout mouse embryos and Nfatc2 −/− ; Nfatc 3 −/− ; Nfatc4 −/− triple-knockout mouse embryos exhibit cardiac development defects similar to those seen in DS, and Nfatc2 −/− ; Nfatc4 −/− double-knockout mice show decreased muscular strength, increased sociability and decreased anxiety-related behaviour that are similar to those seen in DS. Transgenic mouse models and computational simulation have predicted that a 1.5-fold increase of Dyrk1A activity, synergistically acting with another DSCR gene, DSCR1 , would downregulate the activity of the calcineurin/NFAT signalling pathway, thereby inducing the DS-like phenotype [22] . Nevertheless, the exact role of the skewed NFAT pathway in real DS individuals is still debated [8] , and further studies are warranted because the transgenic mice may not always mimic the endogenous levels of overexpressed genes, as they are not subjected to transcriptional and alternative splicing regulations. Interestingly, mice that have only one copy of Dyrk1A through targeted disruption of Dyrk1A in one allele (Dyrk1A +/− mice) also show profound phenotypic abnormalities, including reduced viability, smaller body size, disproportionate decrease in the size of the midbrain and hindbrain regions, changes in pyramidal cell structure and neuromotor and cognitive impairment [23] , [24] , [25] , [26] . The mice homozygous for targeted disruption of Dyrk1A (Dyrk1A −/− -null mice) are embryonic lethal and died between E10.5 and E13.5 [23] . Together, these findings demonstrate that Dyrk1A has distinctively strong dose effects, and that either an excess or a deficit of the kinase activity is detrimental for the normal functioning of the brain and the body. The dose-sensitive nature of Dyrk1A function calls for the development of a method to deliberately manipulate Dyrk1A activity in vivo in order to define its functions and its precise role in DS pathology. Here, we report the development of INDY, a novel potent inhibitor of Dyrk1A. INDY is a highly selective inhibitor of Dyrk1A and is capable of manipulating the activity levels of the kinase in cultured cells and Xenopus embryos. The discovery of INDY would provide a valuable tool for the research of Dyrk1A-related diseases including DS, and may lead to invention of a novel therapeutic strategy for the diseases. Discovery of a novel Dyrk/Clk dual inhibitor INDY To develop a potent inhibitor of Dyrk1A, we screened our compound library. The compound with the strongest inhibition was (1 Z )-1-(3-ethyl-5-hydroxy-2(3 H )-benzothiazoylidene)-2-propanone, which we referred to as INDY (inhibitor of Dyrk), and which showed an half-maximal inhibitory concentration (IC 50 ) of 0.24 μM ( Fig. 1a ). Although INDY shared the benzothiazole structure with the previously reported Clk (cdc2-like kinase) inhibitor, TG003 (refs 27 , 28 ) ( Supplementary Fig. S1 ), it was threefold more potent in inhibiting Dyrk1A compared with TG003 (IC 50 =0.93 μM). The double-reciprocal Lineweaver–Burk plot showed that INDY competitively inhibits Dyrk1A against ATP (Michaelis constant, K m =37 μM) with a K i (inhibition constant) value of 0.18 μM ( Fig. 1b ). INDY also inhibited Dyrk1B, the closest Dyrk kinase family member to Dyrk1A, with an IC 50 of 0.23 μM. In an in vitro assay screening using a panel of 66 protein kinases, INDY (10 μM) showed >90% inhibition on DYRK2, DYRK3 and four other kinases, namely CLK1, CLK4, casein kinase 1 (CSNK1D) and PIM1 ( Supplementary Table S1 ). Harmine, a plant alkaloid, is the most potent Dyrk1A inhibitor reported to date (IC 50 =0.03–0.08 μM) [29] , [30] . Inhibition of Dyrk1A by INDY was comparable with that by harmine ( Supplementary Fig. S1 ), which showed a higher IC 50 (0.35 μM) in our assay compared with the past reports, presumably owing to the different experimental conditions. Interestingly, harmine also inhibited Clks at a level comparable with the inhibition by INDY ( Supplementary Table S2 ), implying a similar structural mechanism of inhibitory action. In addition to inhibiting kinases, harmine also inhibits monoamine oxidase (MAO) A at a considerably lower dose (IC 50 =5 nM) than required for inhibiting Dyrk and Clk family kinases [31] . INDY, however, was substantially free of MAOA inhibitory activity ( Fig. 1c ), which was in sharp contrast to harmine and suggested that there was a biologically significant difference between these compounds. 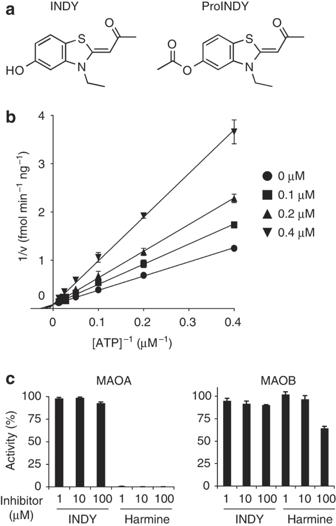Figure 1: Identification of INDY as a Dyrk1A inhibitor. (a) Structures of INDY and proINDY. (b) Double-reciprocal plots of the inhibitory activity of INDY. Dyrk1A kinase activity was measured at the indicated concentrations of INDY and ATP in triplicate. The reciprocal velocity was plotted versus 1/[ATP].Km=37 μM,Vmax=12 fmol min−1ng−1andKi=0.18 μM. Error bars are the standard deviation. (c) Monoamine oxidase (MAO) inhibition by INDY and harmine. MAO activity was measured with an assay based on luminogenic MAO substrate. The percent activities of MAOA or MAOB in the presence of the indicated concentrations of compounds were measured in triplicate. Error bars are the standard deviation. Figure 1: Identification of INDY as a Dyrk1A inhibitor. ( a ) Structures of INDY and proINDY. ( b ) Double-reciprocal plots of the inhibitory activity of INDY. Dyrk1A kinase activity was measured at the indicated concentrations of INDY and ATP in triplicate. The reciprocal velocity was plotted versus 1/[ATP]. K m =37 μM, V max =12 fmol min −1 ng −1 and K i =0.18 μM. Error bars are the standard deviation. ( c ) Monoamine oxidase (MAO) inhibition by INDY and harmine. MAO activity was measured with an assay based on luminogenic MAO substrate. The percent activities of MAOA or MAOB in the presence of the indicated concentrations of compounds were measured in triplicate. Error bars are the standard deviation. Full size image X-ray crystallographic study of the Dyrk1A/INDY complex To determine how INDY inhibits Dyrk1A, we co-crystallized the Dyrk1A/INDY complex and determined its structure by X-ray crystallography. The overall fold of Dyrk1A was similar to those of many other protein kinases reported to date ( Fig. 2a , Supplementary Table S3 ). A biochemical study [32] had shown that Tyr321, which is the second tyrosine of the Tyr-Xaa-Tyr motif in the activation loop, is autophosphorylated. The crystal structure clearly shows the phosphate group on Tyr321, which directly interacts with two arginine residues, Arg325 and Arg328 ( Fig. 2a ). This geometry is almost identical to that found in Erk2, where the phosphorylated tyrosine, Tyr185, is recognized by Arg189 and Arg192 [33] . In the case of Erk2, the phosphorylations of Thr183 and Tyr185 induce a conformational change that creates the P+1 site near Tyr185 for the substrate peptide. Considering that the structure of Dyrk1A around the phosphotyrosine is very similar and that both Erk2 and Dyrk1A prefer a proline residue at the P+1 residue of the substrates, the phosphorylation of Tyr321 is also likely to enhance the activity by formation of the P+1 pocket. 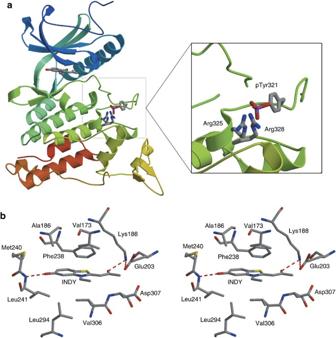Figure 2: Crystal structure of the Dyrk1A/INDY complex. (a) The overall structure. Dyrk1A is shown in ribbon mode. Left, the inhibitor INDY, as well as phosphorylated tyrosine (Tyr321) and two arginine residues that interact with the phosphate group (Arg325 and Arg328) are shown in stick models; right, Tyr321, Arg325 and Arg328 are depicted in a magnified view. (b) Stereoviews of the inhibitor-binding site of the Dyrk1A/INDY complex. The red dotted lines indicate hydrogen bonds. Figure 2: Crystal structure of the Dyrk1A/INDY complex. ( a ) The overall structure. Dyrk1A is shown in ribbon mode. Left, the inhibitor INDY, as well as phosphorylated tyrosine (Tyr321) and two arginine residues that interact with the phosphate group (Arg325 and Arg328) are shown in stick models; right, Tyr321, Arg325 and Arg328 are depicted in a magnified view. ( b ) Stereoviews of the inhibitor-binding site of the Dyrk1A/INDY complex. The red dotted lines indicate hydrogen bonds. Full size image INDY binds to Dyrk1A at the ATP-binding cleft and makes extensive hydrophobic interactions with Val173, Ala186, Phe238, Leu241, Leu294 and Val306 ( Fig. 2b , Supplementary Fig. S2 ). The two polar groups of INDY pin the position of the ligand by two hydrogen bonds: the phenolic hydroxyl group to the main chain nitrogen of Leu241 and the carbonyl oxygen to the side-chain amino group of Lys188, which also forms a salt bridge with Glu203 ( Fig. 2b , Supplementary Fig. S2 ). We also prepared and analysed the Dyrk1A/harmine co-crystal and found that harmine binds to Dyrk1A at the same site in a very similar manner ( Supplementary Fig. S3 ). Most of the hydrophobic interactions as well as two crucial hydrogen bonds are conserved, which probably accounts for the similar affinity of these compounds to Dyrk1A. In-cell inhibition of Dyrk1A by INDY We then asked whether INDY could inhibit Dyrk1A in living cells. The microtubule-associated protein-tau is a well-characterized substrate of Dyrk1A [11] , [34] . Dyrk1A phosphorylates the tau-protein at Thr212, and this phosphorylation event has been observed in the brains of animal models of DS [11] , [34] , [35] . When EGFP-tau was co-transfected with EGFP-Dyrk1A in COS7 cells, the phosphorylated form of EGFP-tau was detected by a phospho-Thr212-specific antibody. This signal declined by addition of INDY in a dose-dependent fashion, showing its potent Dyrk1A-inhibitory effect ( Fig. 3 ). A mild inhibition of tau-phosphorylation was observed at 3 μM, and nearly complete inhibition was seen at 30 μM. 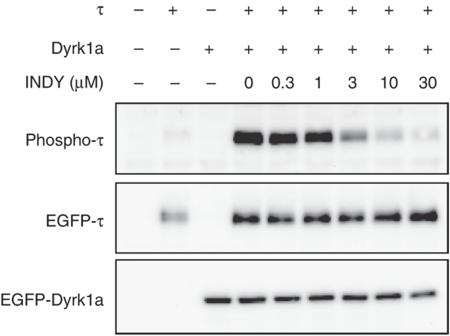Figure 3: Inhibition of Dyrk1A kinase activity by INDY in live cells. COS7 cells were transfected with either EGFP-Dyrk1A and EGFP-tau or both. Transfected cells were treated with the indicated dose of INDY or vehicle alone. Dyrk1A-dependent phosphorylation of Thr212 of EGFP-tau was detected by a phospho-specific antibody. Figure 3: Inhibition of Dyrk1A kinase activity by INDY in live cells. COS7 cells were transfected with either EGFP-Dyrk1A and EGFP-tau or both. Transfected cells were treated with the indicated dose of INDY or vehicle alone. Dyrk1A-dependent phosphorylation of Thr212 of EGFP-tau was detected by a phospho-specific antibody. Full size image Recovery of repressed calcineurin/NFAT signalling As misregulation of calcineurin/NFAT signalling induced DS-like manifestations in transgenic mice [22] , an event that may also result from excessive activity of Dyrk1A, we asked if INDY is capable of modifying the calcineurin/NFAT system. NFATc transcription factors reside in the cytosol of unstimulated cells as phosphorylated proteins. On elevation of cellular Ca 2+ levels, the Ca 2+ -dependent protein phosphatase calcineurin dephosphorylates NFATc, resulting in nuclear transport of NFATc [36] . In the nucleus, NFATc forms a transcription complex with its partner proteins NFATn and binds to the promoter regions of their target genes to initiate the expression [36] . Dyrk1A rephosphorylates nuclear NFATc and works as a priming kinase to invite sequential phosphorylation by glycogen synthase kinase 3, ultimately leading to cytosolic export of NFATc and termination of the expression of the target genes [22] , [37] . We therefore assayed the effect of INDY on the calcineurin/NFAT pathway by imaging the translocation of the EGFP–NFATc1 fusion protein. EGFP–NFATc1 predominantly stayed in the cytosol when expressed in HEK293 cells ( Fig. 4a , top left). On addition of the calcium ionophore ionomycin (IM) to the cells, EGFP–NFATc1 accumulated in the nucleus ( Fig. 4a , top middle). Co-transfection of the Dyrk1A expression vector blocked the nuclear accumulation of EGFP–NFATc1, consistent with its negative regulatory role in the calcineurin/NFAT pathway ( Fig. 4a , bottom left). INDY effectively worked to relocate EGFP–NFATc1 into the nucleus, even in the presence of overexpressed Dyrk1A ( Fig. 4a , bottom right). 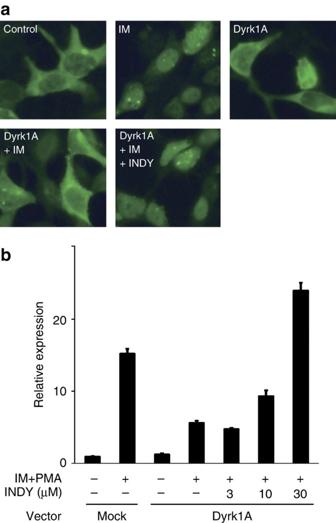Figure 4: Inhibition of the NFAT pathway by Dyrk1A overexpression and its rescue by INDY. (a) Translocation of the EGFP–NFATc1 fusion protein. EGFP–NFATc1 was co-transfected with either Dyrk1A or mock vector into HEK293 cells. Cells were pretreated with INDY (30 μM) or vehicle alone before stimulation with ionomycin (IM; 5 μM). Top left and middle: mock-transfected cells, unstimulated (top left) or IM treated (top middle); top right and bottom: Dyrk1A-transfected cells, unstimulated (top right), IM treated (bottom left) or INDY pre-treated and IM treated (bottom right). (b) Rescue of NFAT-dependent transcription by INDY. The NFAT response element (NFAT-RE)-driven expression of firefly luciferase was measured by a dual luciferase reporter assay. HEK293 cells were transfected with the reporter vectors, and by either Dyrk1A expression vector or empty vector. The cells were treated with IM (5 μM), phorbol 12-myristate 13-acetate (PMA; 10 nM) and the indicated dose of INDY or vehicle alone. The signals were standardized with thymidine kinase (TK) promoter-driven expression ofRenillaluciferase activity. The average ratio (n=3) of NFAT-RE/TK promoter activity was normalized by mock-transfected, unstimulated cells as a control and shown in the graph. Error bars are the standard deviations. Figure 4: Inhibition of the NFAT pathway by Dyrk1A overexpression and its rescue by INDY. ( a ) Translocation of the EGFP–NFATc1 fusion protein. EGFP–NFATc1 was co-transfected with either Dyrk1A or mock vector into HEK293 cells. Cells were pretreated with INDY (30 μM) or vehicle alone before stimulation with ionomycin (IM; 5 μM). Top left and middle: mock-transfected cells, unstimulated (top left) or IM treated (top middle); top right and bottom: Dyrk1A-transfected cells, unstimulated (top right), IM treated (bottom left) or INDY pre-treated and IM treated (bottom right). ( b ) Rescue of NFAT-dependent transcription by INDY. The NFAT response element (NFAT-RE)-driven expression of firefly luciferase was measured by a dual luciferase reporter assay. HEK293 cells were transfected with the reporter vectors, and by either Dyrk1A expression vector or empty vector. The cells were treated with IM (5 μM), phorbol 12-myristate 13-acetate (PMA; 10 nM) and the indicated dose of INDY or vehicle alone. The signals were standardized with thymidine kinase (TK) promoter-driven expression of Renilla luciferase activity. The average ratio ( n =3) of NFAT-RE/TK promoter activity was normalized by mock-transfected, unstimulated cells as a control and shown in the graph. Error bars are the standard deviations. Full size image Because the biological effects of Dyrk1A, such as the maintenance of normal neurological functions, are particularly sensitive to its activity levels, we asked whether INDY could control calcineurin/NFAT signalling in a dose-dependent fashion. For this purpose, we performed a dual luciferase assay to monitor the transcriptional activity that follows NFATc nuclear translocation. Stimulation of HEK293 cells harbouring the NFAT response element (NFAT-RE) reporter vector by IM and phorbol 12-myristate 13-acetate resulted in a 15.2-fold increase of NFAT-RE-driven expression of firefly luciferase. When cells were co-transfected with the Dyrk1A expression vector, the effect of the stimuli was suppressed to only one-third (a 5.7-fold increase) compared with the control ( Fig. 4b ). Addition of 10 μM of INDY partially ameliorated this suppression compared with vehicle alone (a 9.3-fold increase). Treatment with an increased dose (30 μM) of the inhibitor further enhanced the NFAT-RE-dependent transcription and even surpassed the condition under which no exogenous Dyrk1A expression was introduced (a 23.9-fold increase) ( Fig. 4b ). The overriding effect on calcineurin/NFAT signalling seen in high-dose treatment of INDY would be explained by the inhibition of endogenous DYRK family kinases inherent in HEK293 cells [37] . In vivo recovery of Xenopus laevis developmental defects To validate the utility of the Dyrk1A inhibitor on the whole body, we developed a novel in vivo assay. The X. laevis embryo is an ideal platform to observe general effects of Dyrk1A overexpression and to evaluate the effects of inhibitors, because our assay allows relatively good throughput compared with other vertebrate model systems and the consequences can be easily assessed visually [27] . We found a X. laevis cDNA sequence (BC110968, MGC:132284) as well as related EST sequences coding a putative kinase nearly identical to mammalian Dyrk1A from a database search. The kinase, which we named xDyrk1A, showed 92.4, 90.7, 90.2 and 97.5% identity to the Dyrk1A proteins of Homo sapiens, Rattus norvegicus, Mus musculus and X. tropicalis , respectively ( Supplementary Fig. S4 ). When expressed in COS7 cells, the xDyrk1A efficiently phosphorylated tau-proteins and showed sensitivity towards INDY, indistinguishable from its mammalian Dyrk1A counterpart ( Supplementary Fig. S5 ). To investigate the effects of xDyrk1A on the anterior formation, we injected xDyrk1A mRNA into two animal dorsal blastomeres of eight-cell embryos. As a result, deformity was observed in the eye and the head of stage 40/41 tadpoles ( Fig. 5a , top panels), which was accompanied by dorsal deformation in some cases ( Supplementary Fig. S6 ). We introduced a lysine-to-arginine mutation into the kinase catalytic domain of xDyrk1A (xDyrk1A-K180R) to generate its inactive form. Injection of xDyrk1A-K180R mRNA, as well as injection of unrelated control β-globin mRNA, did not cause morphological changes, demonstrating that the deformities were indeed induced by the excessive kinase activity of xDyrk1A ( Fig. 5a , top panels). 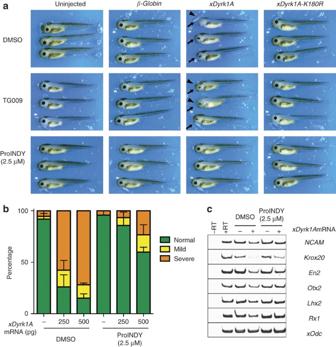Figure 5: Whole-embryo xDyrk1A overexpression assay. (a)In vivorescue of xDyrk1A overexpression-induced deformity.X. laevisembryos were treated with vehicle alone, TG009 (2.5 μM) or proINDY (2.5 μM). The embryos were injected with 500 pg ofβ-globin,xDyrk1Aor kinase-inactivexDyrk1AmRNA (xDyrk-K180R) at the eight-cell stage and incubated until they reached stage 40/41. Arrows, eye deformity; arrowheads, head deformity. (b) Rescue rate of embryo deformity.X. laevisembryos were treated with either proINDY (2.5 μM) or vehicle alone and injected with 250 pg or 500 pg ofxDyrk1AmRNA. Uninjected embryos were used as controls. The percentages of normal embryos, embryos with mild deformity and embryos with severe deformity in each experimental group are depicted in green, yellow and orange, respectively. The embryos were categorized into normal, mild deformity and severe deformity groups according to the degree of eye, head and trunk deformity, as illustrated inSupplementary Figure S6. The mean percentage from two independent experiments and the range for each group are shown. The numbers of embryos used were as follows: for vehicle alone and uninjected: 28 and 37 for the first and second experiments, respectively; vehicle alone and 250 pg mRNA: 35 and 29; vehicle alone and 500 pg mRNA: 41 and 27; proINDY and uninjected: 39 and 35; proINDY and 250 pg mRNA: 23 and 44; and proINDY and 500 pg mRNA: 34 and 29. Error bars indicate the range. (c) Reversal of downregulation of differential neural markers.X. laevisembryos treated with proINDY (2.5 μM) or vehicle alone were injected withxDyrk1AmRNA (500 pg) and grew until stage 17. Expression of depicted differentiation markers was analysed by RT–PCR. xOdc is an internal control. Lanes: −RT, negative control without reverse transcriptase; +RT, uninjected and non-treated. Figure 5: Whole-embryo xDyrk1A overexpression assay. ( a ) In vivo rescue of xDyrk1A overexpression-induced deformity. X. laevis embryos were treated with vehicle alone, TG009 (2.5 μM) or proINDY (2.5 μM). The embryos were injected with 500 pg of β-globin , xDyrk1A or kinase-inactive xDyrk1A mRNA ( xDyrk-K180R ) at the eight-cell stage and incubated until they reached stage 40/41. Arrows, eye deformity; arrowheads, head deformity. ( b ) Rescue rate of embryo deformity. X. laevis embryos were treated with either proINDY (2.5 μM) or vehicle alone and injected with 250 pg or 500 pg of xDyrk1A mRNA. Uninjected embryos were used as controls. The percentages of normal embryos, embryos with mild deformity and embryos with severe deformity in each experimental group are depicted in green, yellow and orange, respectively. The embryos were categorized into normal, mild deformity and severe deformity groups according to the degree of eye, head and trunk deformity, as illustrated in Supplementary Figure S6 . The mean percentage from two independent experiments and the range for each group are shown. The numbers of embryos used were as follows: for vehicle alone and uninjected: 28 and 37 for the first and second experiments, respectively; vehicle alone and 250 pg mRNA: 35 and 29; vehicle alone and 500 pg mRNA: 41 and 27; proINDY and uninjected: 39 and 35; proINDY and 250 pg mRNA: 23 and 44; and proINDY and 500 pg mRNA: 34 and 29. Error bars indicate the range. ( c ) Reversal of downregulation of differential neural markers. X. laevis embryos treated with proINDY (2.5 μM) or vehicle alone were injected with xDyrk1A mRNA (500 pg) and grew until stage 17. Expression of depicted differentiation markers was analysed by RT–PCR. xOdc is an internal control. Lanes: −RT, negative control without reverse transcriptase; +RT, uninjected and non-treated. Full size image To rescue the deformity with INDY, we developed its acetylated derivative, which we referred to as proINDY ( Fig. 1a ). ProINDY has an additional acetyl group linked by an ester bond at the phenolic hydroxyl group of INDY that is expected to make the molecule more lipophilic and enhance its cell membrane permeability. Although proINDY itself inhibits Dyrk1A very weakly in vitro (26.1% inhibition at 10 μM), the ester bond is easily hydrolysed by esterases inherent in cells as well as blood plasma, leading to production of the highly active compound identical to INDY ( Supplementary Fig. S7a ). Indeed, in the cultured cells overexpressing Dyrk1A or xDyrk1A, proINDY inhibited the phosphorylation of Thr212 of the tau-protein ( Supplementary Figs S5 and S7b ). ProINDY also rescued the NFAT pathway at the same concentration as did INDY in Dyrk1A-overexpressing cells ( Supplementary Fig. S7c ), confirming the identical Dyrk1A-inhibitory effect. Furthermore, the Xenopus embryo recovered apparently normal development ( Fig. 5a , bottom panels) after treatment with proINDY. This rescue effect was dependent on xDyrk1A-inhibitory activity, because TG009 (ref. 27 ), another benzothiazole derivative that shows virtually no inhibitory effect on Dyrk1A (IC 50 =251 μM), failed to reverse the deformity ( Fig. 5a middle panels). Highlighting the marked efficiency of proINDY, embryos injected with 250 pg of xDyrk1A mRNA were almost completely rescued at the concentration of 2.5 μM; only 26.1% of the tadpoles developed normally when treated with vehicle alone, whereas 85.8% were normal under the presence of proINDY ( Fig. 5b ). ProINDY was also effective when the embryos were injected with a higher dose of xDyrk1A mRNA (500 pg), but with decreased efficiency (15.3% for ProINDY versus 60.0% for the control). These results strongly suggest that increased xDyrk1A activity is causative of the deformity and it can be reversed by addition of proINDY. The relatively low dose of 2.5 μM did not induce apparent toxicity to the injected embryos. Consistent with their morphological change, differential neural markers were downregulated in xDyrk1A-overexpressed tadpoles. In the embryos injected with 500 pg xDyrk1A mRNA, decreased expression of the pan-neural marker NCAM, hindbrain marker Krox20, midbrain marker En2 and forebrain marker Otx2 were observed from reverse transcription PCR (RT–PCR) analysis ( Fig. 5c ). The eye marker genes, Lhx2 and Rx1 , also showed a similar downregulation. Treatment with proINDY recovered, if not completely, the expression of these markers in agreement with their ability to rescue the morphological abnormalities. INDY is a newly developed potent Dyrk1A inhibitor that was capable of manipulating the Dyrk1A activity levels in living cells. The structure of the co-crystal of Dyrk1A and INDY revealed that the drug binds to its target at the ATP-binding site, consistent with its ATP-competitive nature. ProINDY, an acetylated INDY, worked as a prodrug, which was hydrolysed in vivo to generate INDY and restored the abnormal development of X. laevis tadpoles induced by xDyrk1A mRNA injection into morphologically normal tadpoles. To our knowledge, harmine is the most potent inhibitor of Dyrk1A known to date, and has the advantage of highly selective kinase specificity. It is, however, also a strong MAOA inhibitor and a hallucinogenic central nervous system stimulant [38] , [39] . INDY showed comparable inhibitory potency and similar substrate selectivity with harmine, but had the unique advantage that it did not inhibit MAOA. To explain this selectivity of INDY, the structure of the MAOA/harmine complex [40] (PDB code 2Z5X ) was superimposed on the Dyrk1A/harmine complex using the coordinates of harmine ( Supplementary Fig. S8 ). The Dyrk1A/INDY complex was further superimposed on the Dyrk1A/harmine complex using the coordinates of the protein. The hypothetical MAOA/INDY complex suggests that, although INDY could reproduce many hydrophobic interactions between harmine and MAOA, the N -ethyl group of INDY would collide with Asn181 or Phe208. The inhibitor-binding site of MAOA is a cavity, whereas that of Dyrk1A is a cleft. INDY, which is slightly larger than harmine, can be accommodated in Dyrk1A but not in MAOA. The hypothetical complex also indicated that the terminal methyl group of the propanone moiety of INDY would disturb a network of water-mediated hydrogen bonds of MAOA, which would be energetically unfavourable ( Supplementary Fig. S8 ). Thus INDY and its prodrug form proINDY would be ideal tools that could be substituted for harmine in DS studies and other neuroscience studies concerned with Dyrk1A. Other commonly used Dyrk1A inhibitors include roscovitine, purvalanol A and epigallocatechin gallate (EGCG) [41] . Roscovitine and purvalanol A are several-fold more potent inhibitors of cyclin-dependent kinases compared with Dyrk1A [41] , and thus their use may be limited because of their effects on the cell cycle. EGCG, a catechin found in green tea, also inhibited Dyrk1A, but its profound promiscuity may also hamper the elucidation of its effect on Dyrk1A. EGCG is a strong anti-oxidant and a metal chelator; it is known to inhibit proteasome, matrix metalloproteinase, dihydrofolate reductase, DNA methyltransferase, topoisomerase II and telomerase; it also binds to laminin receptor, DNA and RNA [42] , [43] . Thus, EGCG has a profound influence on many signalling pathways, such as those mediated by protein kinase C, nuclear factor-κB, epidermal growth factor receptor, mitogen-activated protein kinases, activator protein 1 transcription factor and hypoxia-inducible factor 1 [42] , [43] . For all these reasons, we concluded that INDY is a novel potent Dyrk1A inhibitor with unique characteristics different from its previously known counterparts. In addition to Dyrk1A, INDY and harmine inhibit other Dyrk family members, including DYRK1B, DYRK2, DYRK3 and DYRK4, as well as Clk family kinases ( Supplementary Tables S1 and S2 ). To the best of our knowledge, there are no reports of abnormal phenotypes or pathological conditions that are derived from deficiency of other DYRK and Clk family kinases. DYRK1B (also known as Mirk) is reported to be involved in muscle differentiation, although its knockout mouse was reportedly viable [44] . The apparently normal morphology of X. laevis embryos treated with proINDY suggests that the moderate reduction of the activities of these kinases might be well tolerated. In the case of DS pathogenesis, a 1.5-fold increase of Dyrk1A expression is considered to be pathogenic [14] , [15] , [16] , [17] , [18] , [22] . It is possible that the use of a relatively mild dose of INDY that would simply reduce its activity to the original level might not elicit critical off-target effects. Nevertheless, contributions from the effects of Clk family kinase inhibition should always be considered when interpreting the biological effects of INDY. The xDyrk1A overexpression assay using X. laevis embryos enabled assessment of the in vivo benefit of inhibitors. This method is unique in that it allows an in vivo assay at a level of whole vertebrate development while also allowing a relatively high throughput. We consider that this whole-embryo assay would be a valuable tool in the further search for and refinement of Dyrk1A inhibitors. On the other hand, we are aware that this assay monitors an artificial phenotype that does not necessarily reflect bona fide DS pathology, making it unsuitable for detailed study of the molecular pathogenesis of DS. At present, the downstream events of xDyrk1A overexpression that lead to the downregulation of differentiation markers and head/eye deformity are unknown. It may be noted that Krox20, one of the downregulated markers, has been reported to be a downstream target of NFAT pathways in mammalian brain development [45] . It would be interesting to examine whether the administration of INDY could rescue the phenotypes of Dyrk1A-transgenic mice or the phenotypes of other mice models of human chromosome 21 trisomy, because such an experiment would elucidate the role of Dyrk1A in DS pathogenesis and demonstrate the possible utility of Dyrk1A inhibitors as DS therapeutic agents. Previous reports demonstrated that transgenic mice carrying a yeast artificial chromosome containing Dyrk1A were rescued from neurological defects when they were fed with green tea daily [46] . This effect may be attributed to EGCG, which is present in high concentrations in green tea leaves. In another report, treatment of Dyrk1A-transgenic mice by harmine reversed the decreased plasma homocysteine levels caused by excess Dyrk1A activity [47] . INDY may provide similar rescue effects on DS model mice. It must be noted, however, that the interpretation of drug effects is often difficult in model animals of contiguous genetic syndromes such as DS. Because of the complex interactions between the human chromosome 21 genes, manipulation of a gene activity may affect the activities of other genes and lead to an unpredicted outcome [48] . Such an effect may also occur in the case of Dyrk1A. Several mouse models that overexpress Dyrk1A through yeast artificial chromosome clones, bacterial artificial chromosome clones or exogenous promoters exhibit neurobehavioral abnormalities [14] , [15] , [16] , [17] , [18] , [19] , [20] , [21] . However, in the case of Ts1Rhr mice, trisomy of a genetic segment that contains 33 genes including Dyrk1A was not sufficient to induce neurobehavioral phenotypes [9] . Nonetheless, the gene segment amplified in Ts1Rhr was indispensable for the neurobehavioral abnormalities of Ts65Dn, a DS model mouse that harbours a trisomy of an overlapping genetic segment that is longer than that of Ts1Rhr [9] . The exact role of Dyrk1A in DS would be defined in the context of its complete trisomy, and further development of an improved DS model mice would present more relevant tools for this purpose [49] . We are currently studying the pharmacological effect of INDY in several DS model mice. Furthermore, excessive Dyrk1A activity may be pivotal to the pathogenesis of Alzheimer's disease (AD) and other tauopathies. Recent studies have highlighted the role of Dyrk1A as the priming kinase of multiple phosphorylation of the tau-protein. In vitro experiments showed that when the tau-protein was phosphorylated at Thr212 by Dyrk1A, it became prone to phosphorylation by other kinases including GSK3β, at multiple sites, leading to pathogenic aggregation of the protein and formation of neurofibrillary tangles [11] , [34] , [35] . Studies of the brains of patients with AD revealed increased expression of Dyrk1A in both the brains and the specific neurons affected by tau-aggregation [13] , [50] , [51] . These findings are further reinforced by the fact that DS is strongly associated with early-onset AD [2] , [4] . Nearly all individuals with DS develop the typical AD histopathology of neurofibrillary tangles and amyloid plaques when they are above the age of 30 years [52] , and between 50 and 70% of DS individuals develop dementia by the age of 60 years [2] , [4] . Because INDY inhibited Thr212 phosphorylation under experimental conditions, it would serve as a useful tool in investigating the role of Dyrk1A in tau-aggregate formation and thus could be used to examine the possibility that Dyrk1A might be a novel drug target of AD and other tauopathies. Synthesis of inhibitors INDY and proINDY were prepared using standard synthetic procedures from TG003 (ref. 27 ), as described in the Supplementary Methods . Cell culture HEK293 and COS7 cells were cultured in Dulbecco's modified Eagle's medium containing 10% fetal calf serum. For transfection of plasmids, GeneJuice Transfection Reagent (Merck) or FuGene HD Transfection Reagent (Roche Applied Science) was used according to the manufacturer's instructions. Plasmid construction and mRNA synthesis EGFP-Dyrk1A and pGEX-2TK-DYRK1B were kind gifts from Professor Dr Walter Becker (Institute for Pharmacology and Toxicology) [1] , [53] . The Dyrk1A cDNA was amplified and a FLAG epitope tag was added to its C-terminus by PCR. The PCR fragment was subcloned into pCS2+ vector to generate the FLAG-Dyrk1A expression vector. For expression of the recombinant Dyrk1A kinase domain in Escherichia coli , a cDNA fragment encoding the kinase domain (amino acids 126–490) of human Dyrk1A was generated. The fragment was joined with the TEV protease cleavage site directly upstream of the start codon and subcloned into the pET28 vector. To generate the EGFP-tau expression vector, the human MAPT cDNA (NM_016834) was obtained by RT–PCR from mRNAs of human neuroblastoma SH-SY5Y cells and the PCR fragment was introduced into the pEGFP-C1 plasmid. For construction of the expression vector for the EGFP–NFATc1 fusion protein, cDNA fragments coding EGFP and human NFATc1 (BC112243.1, obtained from Thermo Scientific) were amplified by PCR. The fragments were simultaneously subcloned into a pcDNA3 expression vector (Invitrogen) harbouring att R1 and att R2 sites using a Multisite Gateway Pro Plus kit (Invitrogen). For expression of xDyrk1A, a cDNA fragment of xDyrk1A (MGC:132284, obtained from Thermo Scientific) was amplified by RT–PCR, joined with a N-terminal FLAG epitope tag and subcloned into the pCS2+ vector to generate the FLAG-xDyrk1A plasmid. To generate a kinase-inactive mutant of xDyrk1A, Lys180 of xDyrk1A, which corresponds to Lys188 of human Dyrk1A, was replaced with Arg (xDyrk1A-K180R) by using a QuickChange II XL Site-directed Mutagenesis Kit (Stratagene) according to the manufacturer's instructions. The primers used for mutagenesis were as follows: sense 5′-GTGGGTGGCGATTAGAATTATAAAGAACAAG-3′ and antisense 5′-CTTGTTCTTTATAATTCTAATCGCCACCCAC-3′. For preparation of xDyrk1A and xDyrk1A-K180R mRNAs, capped mRNAs were synthesized from linearized vectors with an mMessage mMachine Kit (Ambion) using the FLAG-xDyrk1A plasmid as a template. Determination of IC 50 values against Dyrk1A and Dyrk1B The Dyrk1A in vitro kinase assay was performed as described previously [27] , with minor modifications. Human recombinant Dyrk1A was purchased from Invitrogen. GST-fused human Dyrk1B was expressed in E. coli and purified with glutathione Sepharose. The kinase activities of Dyrk1A and Dyrk1B were assayed in a reaction mixture containing serially diluted inhibitors, 10 mM MOPS-KOH (pH 7.0), 10 mM magnesium acetate, 200 μM EDTA, 10 μM ATP, 4 μCi [γ- 32 P]ATP, 31 μg human myelin basic protein (Millipore) and 0.1–1 μg recombinant Dyrk1A or Dyrk1B in a final volume of 25 μl. The final concentration of DMSO was adjusted to 1%, regardless of the inhibitor concentration. The reaction mixture was incubated at 30 °C for 10 min and 15 μl of the reaction was spotted onto P81, a phosphocellulose membrane (Whatman). The kinase assay conditions, including the incubation period and concentration of kinases and substrates, were optimized to maintain linearity during incubation. The membrane was washed with 5% phosphoric acid solution for at least 15 min. The radioactivity was measured using a liquid scintillation counter. The net radioactivity was deduced by subtracting the background count from the reaction mixture without kinase, and the data are expressed as the percentage to the control sample containing the solvent. As for determination of Dyrk1A inhibition by proINDY at a single concentration of 10 μM, the recombinant human Dyrk1A (amino acids 126–490) was used to phosphorylate myelin basic protein substrate. Lineweaver–Burk plot To obtain a Lineweaver–Burk plot, the bacterially expressed human Dyrk1A kinase domain (amino acids 126–490) was purified with Ni-NTA agarose. The kinase reaction was performed by essentially the same method as described for the IC 50 determination, with the difference that 80 ng of purified kinase and 2 μg of synthetic RS peptide [54] (NH 2 -RSPSYGRSRSRSRSRSRSRSRSNSRSRSY-OH) were used in the assay. The K m , K i and V max (concentration of substrate) values were calculated with Prism5 software (GraphPad Software) using the competitive inhibition model. Single-concentration kinase inhibition All kinases were assayed at an inhibitor concentration of 10 μM and an ATP concentration of 10 μM unless otherwise noted. Radioisotope-based assays were performed for ASK1, DYRK1B, DYRK2, CSNK1D, CLK4, GSK3α, GSK3β, HIPK1 and MET, using essentially the same technique as described above. Other kinases were assayed by the SelectScreen Kinase Profiling Service (Invitrogen; see Supplementary Tables S1 and S2 ). Detailed assay conditions for each kinase are described in the Supplementary Methods . MAO assay The MAO inhibitory activities of INDY and harmine were measured by an MAO-Glo Assay System (Promega) using human recombinant MOA-A and MOA-B (both from Sigma-Aldrich) according to the manufacturer's instructions. In-cell phosphorylation assay COS7 cells were co-transfected with EGFP-tau and either FLAG-Dyrk1A or FLAG-xDyrk1A expression vector. At 4 h after transfection, the cells were treated with the indicated amounts of inhibitors and further incubated for 20 h. Then, the cells were lysed and analysed by western blotting using anti-phosphorylated-tau (pT212) antibody (Biosource), anti-EGFP antibody (Medical & Biological Laboratories) or anti-FLAG antibody (Sigma-Aldrich). X-ray crystallography The kinase domain (amino acids 126–490) of human Dyrk1A with an N-terminal histidine tag was expressed in E. coli and first purified with Ni-NTA agarose. After the removal of the histidine tag with AcTEV protease (Invitrogen), the protein was further purified with ion-exchange chromatography and size-excision chromatography. Then, the protein was concentrated to 5.0 mg ml −1 in 50 mM Tris–HCl (pH 8.0), 100 mM NaCl, 2 mM dithiothreitol, 50 mM arginine, 50 mM glutamic acid and 10% glycerol before crystallization. The crystals of Dyrk1A were obtained with the hanging-drop method at 20 °C, using reservoirs containing 0.1 M sodium cacodylate (pH 6.5), 0.2 M sodium acetate, 30% polyethylene glycol 4000 and 0.5 mM inhibitor (INDY or harmine). The asymmetric unit contained four copies of Dyrk1A/inhibitor complexes. The diffraction data were collected at photon factory beamline NW12A at 100 K and processed with HKL2000 (HKL Research). The structure was solved by molecular replacement with a model based on the crystal structure of Clk1 (PDB entry code 1Z57 ) using the program Phaser [55] , and refinement was performed with the CNS suite [56] . Restraints over non-crystallographic symmetry were applied during the refinement. The crystallographic statistics are summarized in Supplementary Table S3 . The coordinates and structure factors are in preparation for deposition to the protein data bank. During the course of our study, the crystal structures of Dyrk1A in different space groups have been deposited in the protein data bank (PDB code 2VX3 and 2WO6 ). EGFP–NFAT localization assay HEK293 cells were grown on coverslips coated with atelocollagen (Koken) and transfected with EGFP–NFATc1-expressing vector. On the next day, the cells were pre-treated with inhibitors (30 μM) for 3 h and then stimulated with IM (5 μM) for 1 h. Cells were fixed and observed for fluorescence. Dual luciferase reporter assay The dual luciferase reporter assay was performed using a Dual-Luciferase Reporter Assay System (Promega) according to the manufacturer's instructions. NFAT transcriptional activity in the cells was monitored with a pGL4.30[luc2P/NFAT-RE/Hygro] vector (Promega) that contained an NFAT-RE to drive the expression of the firefly luciferase reporter gene. The pRL-TK vector, which expresses Renilla luciferase under the herpes simplex virus thymidine kinase promoter, was co-transfected as an internal control. HEK293 cells were transfected with the FLAG-Dyrk1A vector and reporter vectors. The next day, cells were treated with IM (2.5 μM) and phorbol-12-myristate-13-acetate (10 nM) along with the indicated amounts of inhibitors. Cells were further incubated for 8 h and then cell lysates were harvested to measure the luciferase activity. Hydrolysis of proINDY and HPLC analysis Inhibitors were mixed with rat plasma at a concentration of 100 μM and immediately extracted with acetonitrile. The sample was analysed by HPLC using a COSMOSIL ODS column (250×4.6 mm; Nacalai Tesque), with a mobile phase of 0–80% aqueous acetonitrile at 40 °C, and monitored by absorbance at 356 nm. Handling of the X. laevis embryos and RT–PCR analysis xDyrk1A and xDyrk1A-K180R mRNAs were injected into two animal dorsal blastomeres at the eight-cell-stage embryos for RT–PCR analysis and observation of embryo phenotypes. The solutions including proINDY or TG009 (2.5 μM each) were used for treating embryos just after microinjection. The head regions of the injected embryos were dissected at the neural stage (stage 17), and total RNAs were prepared using TRIzol (Invitrogen). cDNA synthesis was carried out using Moloney murine leukaemia virus reverse transcriptase (Invitrogen). The sequences of the primer pairs were as described previously [57] , [58] . How to cite this article: Ogawa, Y. et al . Development of a novel selective inhibitor of the Down syndrome-related kinase Dyrk1A. Nat. Commun. 1:86 doi: 10.1038/ncomms1090 (2010).